Neuron-released oligomeric α-synuclein is an endogenous agonist of TLR2 for paracrine activation of microglia Abnormal aggregation of α-synuclein and sustained microglial activation are important contributors to the pathogenic processes of Parkinson’s disease. However, the relationship between disease-associated protein aggregation and microglia-mediated neuroinflammation remains unknown. Here, using a combination of in silico , in vitro and in vivo approaches, we show that extracellular α-synuclein released from neuronal cells is an endogenous agonist for Toll-like receptor 2 (TLR2), which activates inflammatory responses in microglia. The TLR2 ligand activity of α-synuclein is conformation-sensitive; only specific types of oligomer can interact with and activate TLR2. This paracrine interaction between neuron-released oligomeric α-synuclein and TLR2 in microglia suggests that both of these proteins are novel therapeutic targets for modification of neuroinflammation in Parkinson’s disease and related neurological diseases. The role of innate immune responses of microglia in neurodegenerative processes in many central nervous system diseases has become increasingly evident [1] , [2] , [3] . Abnormal accumulation of specific protein aggregates in neurons and glia is another common pathological feature shared by most neurodegenerative diseases. Whether these two events are related, and, if so, how misfolding and aggregation of specific proteins in neurons might influence the inflammatory milieu in brain parenchyma remains unknown. A neuronal protein, α-synuclein, has been implicated in many neurodegenerative diseases, including Parkinson’s disease (PD), dementia with Lewy bodies, multiple system atrophy and a Lewy body variant of Alzheimer’s disease (AD) [4] . Although it is a typical cytosolic protein, a small amount of α-synuclein can be released from neurons via brefeldin A-insensitive, unconventional exocytosis [5] , [6] . The structure of the released α-synuclein is unknown. However, there is evidence to suggest that misfolding and aggregation facilitate the release of this protein from neuronal cells [5] . Released α-synuclein can be transferred to neighbouring neurons and astroglia, promoting formation of inclusion bodies and inducing cell death in neurons and proinflammatory responses from astroglia [7] , [8] . In the present study, we attempted to determine the role of neuron-released α-synuclein in microglial activation, the major culprit of inflammation in brain parenchyma, and the mechanism underlying this process. Cell-released α-synuclein induces microglia activation We collected culture media from differentiated SH-SY5Y cells (dSY5Y) overexpressing either human α-synuclein (αSCM) or β-galactosidase (LZCM) ( Supplementary Fig. S1a ). We chose LacZ gene because it is not a mammalian gene and, thus, it is unlikely to produce unwanted complications, and because among the control genes we tested, only LacZ showed expression levels higher than those of α-synuclein. Ectopic expression of these genes did not affect the viability of dSY5Y cells ( Supplementary Fig. S2 ). The concentrations of α-synuclein in the αSCM were determined by enzyme-linked immunosorbent assay (ELISA), and the measurements resulted in an average of 1.06±0.371 μg ml −1 ( Supplementary Fig. S1b ). These media were applied to primary rat microglia at a concentration of 0.1–5.3 μg ml −1 α-synuclein. Microglia treated with αSCM, but not with LZCM, underwent a series of changes indicating proinflammatory activation, including increased morphological changes to amoeboid shapes increased, production of nitric oxide and intracellular reactive oxygen species, increased proliferation and increased production of proinflammatory cytokines at the levels of both messenger RNA and secreted protein ( Fig. 1a–f ). Contamination of adenoviral vectors in αSCM has been ruled out ( Supplementary Fig. S3 ). Induction of cytokine production was gradually reduced by serial depletion of α-synuclein proteins from the conditioned medium ( Fig. 1g ), while α-synuclein proteins purified from αSCM induced cytokine production in a dose-dependent manner ( Fig. 1h ). From these results, we conclude that α-synuclein released from neuronal cells induces proinflammatory responses from microglia. 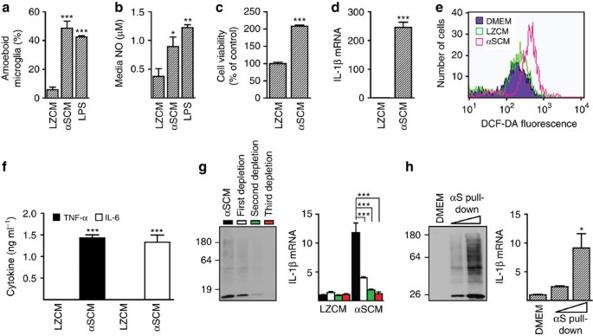Figure 1: dSY5Y-released α-synuclein activates microglia. Rat primary microglia was treated with LZCM, αSCM or lipopolysaccharide (1 μg ml−1, a positive control) for the indicated hours. Lipopolysaccharide is an endotoxin that activates microglial responses that we tested, and therefore, was used as a positive control. (a) Percentage of microglial cells with amoeboid morphology (n=6). (b) Nitric oxide produced from microglia (n=5). (c) Microglial proliferation (n=6). (d) Relative expression of IL-1β mRNA. Real-time PCR data were normalized with the average value of LZCM (n=3). (e) Quantification of intracellular reactive oxygen species levels using flow cytometry. This is the representative result of three independent experiments. (f) Quantification of cytokines using ELISA in the microglial culture media (n=3). (g) Depletion of α-synuclein and microglia activation activity from αSCM. Three successive rounds of depletion were performed using an affinity resin. For cytokine induction (n=3), the amount of α-synuclein in αSCM used was 0.1 μg ml−1. (h) Cytokine induction by his-tagged α-synuclein pulled down from his-αSCM. Western blot shows different amounts of pulled-down α-synuclein used in microglia activation (n=3). Morphology analysis (a), NO production analysis (b), proliferation assay (c), iROS production (e) and cytokine ELISA quantification (f) were performed at 24 h post treatment. Relative mRNA expression (d,g,h) was determined at 2 h post treatment. Morphology analysis (a), NO production analysis (b) and relative mRNA expression (g,h) data were compared by one-way analysis of variance. Proliferation assay (c), cytokine gene expression (d) and cytokine ELISA (f) data were analysed using unpairedt-test. Error bars represent±s.e.m. *P<0.05; **P<0.01; ***P<0.001. ‘n’ represents the number of independent experiments and each experiment was performed at least in triplicate. Figure 1: dSY5Y-released α-synuclein activates microglia. Rat primary microglia was treated with LZCM, αSCM or lipopolysaccharide (1 μg ml −1 , a positive control) for the indicated hours. Lipopolysaccharide is an endotoxin that activates microglial responses that we tested, and therefore, was used as a positive control. ( a ) Percentage of microglial cells with amoeboid morphology ( n =6). ( b ) Nitric oxide produced from microglia ( n =5). ( c ) Microglial proliferation ( n =6). ( d ) Relative expression of IL-1β mRNA. Real-time PCR data were normalized with the average value of LZCM ( n =3). ( e ) Quantification of intracellular reactive oxygen species levels using flow cytometry. This is the representative result of three independent experiments. ( f ) Quantification of cytokines using ELISA in the microglial culture media ( n =3). ( g ) Depletion of α-synuclein and microglia activation activity from αSCM. Three successive rounds of depletion were performed using an affinity resin. For cytokine induction ( n =3), the amount of α-synuclein in αSCM used was 0.1 μg ml −1 . ( h ) Cytokine induction by his-tagged α-synuclein pulled down from his-αSCM. Western blot shows different amounts of pulled-down α-synuclein used in microglia activation ( n =3). Morphology analysis ( a ), NO production analysis ( b ), proliferation assay ( c ), iROS production ( e ) and cytokine ELISA quantification ( f ) were performed at 24 h post treatment. Relative mRNA expression ( d , g , h ) was determined at 2 h post treatment. Morphology analysis ( a ), NO production analysis ( b ) and relative mRNA expression ( g , h ) data were compared by one-way analysis of variance. Proliferation assay ( c ), cytokine gene expression ( d ) and cytokine ELISA ( f ) data were analysed using unpaired t -test. Error bars represent±s.e.m. * P <0.05; ** P <0.01; *** P <0.001. ‘ n ’ represents the number of independent experiments and each experiment was performed at least in triplicate. Full size image Signalling in microglia exposed to cell-released α-synuclein In order to gain a comprehensive understanding of the mechanism of α-synuclein-induced microglial activation, we performed transcriptome analyses using microglial cells treated with either αSCM or LZCM at two different time points, 6 and 24 h. We obtained a total of 2,009 differentially expressed genes (DEGs; 877 DEGs at 6 h only, 797 DEGs at 24 h only, and 335 DEGs common at both time points; Supplementary Fig. S4a ). KEGG pathway-enrichment analyses of upregulated genes showed specific activation of the Jak-STAT signalling pathway during early responses, and leukocyte transendothelial migration, natural killer cell-mediated cytotoxicity and regulation of actin cytoskeleton during late responses (GSE26532, Supplementary Fig. S4b , Supplementary Tables S1 and S2 ). On the other hand, Toll-like receptor (TLR) signalling, cytokine receptor signalling and other immune receptor signalling pathways were activated with high statistical significance at both early and late time points. Using the DEGs involved in these pathways in concert with protein–protein interaction data from public databases, we have constructed a model for a microglial signalling network activated by exposure to dSY5Y-released α-synuclein. According to the model, the TLR2 and cytokine receptor signalling pathways are activated early, producing various proinflammatory cytokines and chemokines. Later, cell migration and actin cytoskeleton rearrangement pathways are activated, while TLR signalling and cytokine/chemokine production are sustained ( Fig. 2a ). Validation of gene expression changes in these signalling pathways was provided by reverse transcriptase PCR ( Fig. 2b ), and activation of the TLR2 downstream signalling pathway was validated by increased IκB degradation and p38 phosphorylation ( Fig. 2c ). 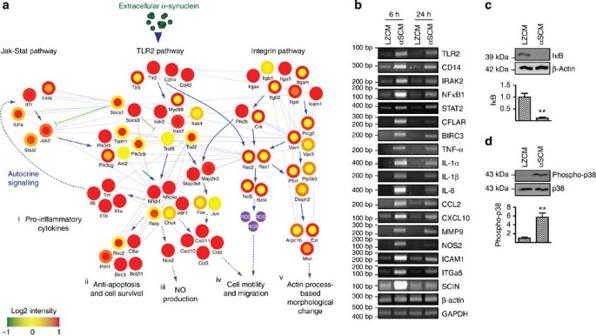Figure 2: Hypothetical signalling network of microglia activated by cell-released α-synuclein. (a) Hypothetical signalling network was constructed by using DEGs from αSCM-exposed microglia. Alterations of gene expression were detected at two different time points (inner circle, 6 h and outer circle, 24 h). (b) Reverse transcriptase PCR analysis of genes identified in the network. (c,d) IκB degradation (c) and phosphorylation of p38 MAP kinase (d) in microglia exposed to αSCM for 15 min (n=4). All data were analysed using unpairedt-test. Error bars represent ±s.e.m. **P<0.01. ‘n’ represents the number of independent experiments. Figure 2: Hypothetical signalling network of microglia activated by cell-released α-synuclein. ( a ) Hypothetical signalling network was constructed by using DEGs from αSCM-exposed microglia. Alterations of gene expression were detected at two different time points (inner circle, 6 h and outer circle, 24 h). ( b ) Reverse transcriptase PCR analysis of genes identified in the network. ( c , d ) IκB degradation ( c ) and phosphorylation of p38 MAP kinase ( d ) in microglia exposed to αSCM for 15 min ( n =4). All data were analysed using unpaired t -test. Error bars represent ±s.e.m. ** P <0.01. ‘ n ’ represents the number of independent experiments. Full size image Role of Tlr2 in α-synuclein-induced microglia activation Involvement of the TLR2 pathway is one of the striking features of the signalling network model. The role of TLRs as modulators in neurological disorders has received increasing recognition. TLR4 and its interaction with extracellular high-mobility group box-1 contribute to generation of seizures [9] . In animal models of stroke, TLR2 and 4 induced proinflammatory reactions resulting in aggravated tissue damage [10] . TLR2 and 4 have been implicated in both clearance of extracellular amyloid β (Aβ) peptide and Aβ-induced microglial activation [11] , [12] , [13] , [14] . Amyloid structure has also been suggested as crucial in triggering of TLR2-mediated inflammatory responses in innate immune cells [15] , [16] . In a rat model, administration of TLR3 agonist into the substantia nigra (SN) induced sustained inflammation and increased susceptibility of dopaminergic neurons to oxidative stress [17] , suggesting that TLR modulation might have therapeutic implications for PD. In order to verify involvement of the TLR system, we examined inflammatory responses to dSY5Y-derived α-synuclein in microglia isolated from mice deficient of Tlr2 , 3 or 4 gene ( Tlr2 −/− , Tlr3 −/− and Tlr4 −/− ). Depletion of Tlr2 gene resulted in complete elimination of cytokine/chemokine gene induction upon exposure to αSCM at both mRNA and protein levels ( Fig. 3a ; Supplementary Figs S5 and S6 ). Treatment with blocking antibody against TLR2 also resulted in elimination of αSCM-induced cytokine gene expression ( Fig. 3c ). In addition, αSCM activated TLR2 signalling cascade in the HEK293 reporter cells (HEK-Blue-TLR2) ectopically expressing human TLR2 and CD14 ( Fig. 3d ). dSY5Y-released α-synuclein proteins purified from the conditioned medium also showed Tlr2 -dependent cytokine production ( Fig. 3e ). Conditioned medium obtained from the wild-type (WT) mouse primary cortical neurons also activated TLR2, whereas that obtained from α-synuclein null mice did not ( Fig. 3f , Supplementary Fig. S7 ). Activation of TLR2 could be observed at concentrations of α-synuclein as low as 1 ng ml −1 in the HEK293 reporter cells ( Supplementary Fig. S8 ), the level comparable to the levels found in the human interstitial fluid [18] ( Supplementary Note 1 ). In contrast, Tlr3 or 4 gene depletion had no effect on α-synuclein-induced gene induction of proinflammatory cytokines/chemokines ( Fig. 3a ). Significant reduction of α-synuclein-induced IκB degradation and p38 phosphorylation was observed in Tlr2 −/− mouse microglia ( Fig. 3g ), confirming that TLR2 mediates α-synuclein-induced signalling in microglia. These results provide validation for the signalling network model in which the TLR2 signalling pathway is specifically involved in the proinflammatory responses of microglia to α-synuclein released from cells, including neurons. 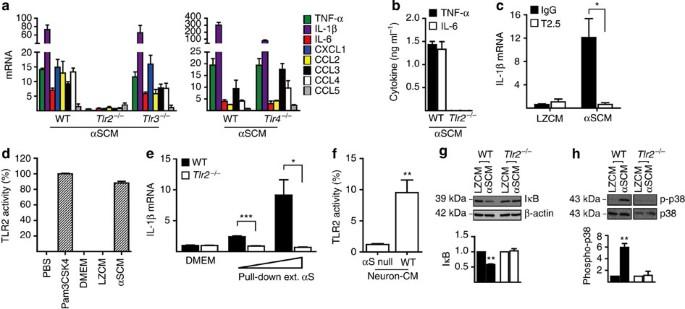Figure 3: Microglia activation by cell-released α-synuclein is mediated by TLR2. (a) Expression of cytokines and chemokines upon treatment of αSCM in WT,Tlr2−/−,Tlr3−/−, andTlr4−/−mouse microglia (n=3). (b) αSCM-induced cytokine production and release in WT andTlr2−/−microglia (n=3). (c) Effects of TLR2-blocking antibody (T2.5) on induction of IL-1β mRNA. Microglia were pre-incubated with either T2.5 or control IgG for 30 min before addition of αSCM or LZCM (n=3). (d) TLR2 activity was determined in the HEK-Blue-TLR2 reporter cells. Pam3CSK4 (10 ng ml−1) is a known TLR2 agonist and used as a positive control (n=3). (e) Induction of IL-1β mRNA by different amounts of α-synuclein purified from αSCM (n=3). (f) TLR2 activation by the endogenous α-synuclein released from mouse primary cortical neurons. Culture media from WT and α-synuclein null mice primary neurons were treated to the HEK-Blue-TLR2 reporter cells (n=3). (g,h) TLR2-dependent IκB degradation (g) and phosphorylation of p38 MAP kinase (h) in microglia exposed to αSCM (n=3). Relative mRNA expressions (a,c,e) were determined at 2 h post treatment. Cytokine ELISA (b) was performed at 6 h post treatment. IκB degradation (g) and p38 phosphorylation (h) analyses were performed at 15 min post treatment. All data were analysed using unpairedt-test. Error bars represent±s.e.m. *P<0.05; **P<0.01; ***P<0.001. ‘n’ represents the number of independent experiments, and each experiment was performed at least in triplicate. Figure 3: Microglia activation by cell-released α-synuclein is mediated by TLR2. ( a ) Expression of cytokines and chemokines upon treatment of αSCM in WT, Tlr2 −/− , Tlr3 −/− , and Tlr4 −/− mouse microglia ( n =3). ( b ) αSCM-induced cytokine production and release in WT and Tlr2 −/− microglia ( n =3). ( c ) Effects of TLR2-blocking antibody (T2.5) on induction of IL-1β mRNA. Microglia were pre-incubated with either T2.5 or control IgG for 30 min before addition of αSCM or LZCM ( n =3). ( d ) TLR2 activity was determined in the HEK-Blue-TLR2 reporter cells. Pam3CSK4 (10 ng ml −1 ) is a known TLR2 agonist and used as a positive control ( n =3). ( e ) Induction of IL-1β mRNA by different amounts of α-synuclein purified from αSCM ( n =3). ( f ) TLR2 activation by the endogenous α-synuclein released from mouse primary cortical neurons. Culture media from WT and α-synuclein null mice primary neurons were treated to the HEK-Blue-TLR2 reporter cells ( n =3). ( g , h ) TLR2-dependent IκB degradation ( g ) and phosphorylation of p38 MAP kinase ( h ) in microglia exposed to αSCM ( n =3). Relative mRNA expressions ( a , c , e ) were determined at 2 h post treatment. Cytokine ELISA ( b ) was performed at 6 h post treatment. IκB degradation ( g ) and p38 phosphorylation ( h ) analyses were performed at 15 min post treatment. All data were analysed using unpaired t -test. Error bars represent±s.e.m. * P <0.05; ** P <0.01; *** P <0.001. ‘ n ’ represents the number of independent experiments, and each experiment was performed at least in triplicate. Full size image Interaction of cell-released α-synuclein with TLR2 Based on the functional significance of TLR2 in α-synuclein-induced microglial activation, we attempted to determine whether TLR2 is the receptor for dSY5Y-released α-synuclein. First, we examined the interaction between dSY5Y-released α-synuclein and TLR2 in the BV2 microglial cell line by assessing the competition between α-synuclein and anti-TLR2 antibody (T2.5). The cells showed robust binding of the TLR2 antibody on the cell surface ( Fig. 4a ; Dulbecco’s modified Eagle’s medium control). However, pretreatment with αSCM resulted in significantly reduced binding of the TLR2 antibody, whereas pretreatment with LZCM had little effect. This result suggests a direct interaction between dSY5Y-released α-synuclein and TLR2, which precludes the interaction of the antibody with TLR2 ( Supplementary Note 2 ). Next, we demonstrated that internalization of externally treated dSY5Y-released α-synuclein into microglia was significantly reduced by Tlr2 gene depletion ( Fig. 4b , Supplementary Fig. S9 ) or by co-treatment with TLR2-blocking antibody ( Fig. 4c ). Internalization was increased upon ectopic expression of TLR2 proteins in COS-7 cells ( Fig. 4d ). In addition, internalized α-synuclein was found to be colocalized with TLR2 in the same internal compartments ( Fig. 4e ). These results demonstrate that TLR2 is the receptor for cell-released extracellular α-synuclein, and that it is responsible not only for signalling and inflammatory responses but also for binding and internalization of this protein. 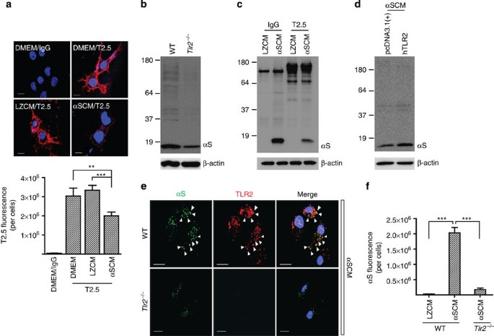Figure 4: Properties of TLR2 as the receptor for cell-released α-synuclein. (a) Competition between TLR2 antibody (T2.5) and dSY5Y-released α-synuclein for binding to the surface of BV2 microglia (n=3). Scale bar, 10 μm. (b) Uptake of α-synuclein by WT andTlr2−/−mouse microglia. Cells were treated with αSCM for 30 min, and then analysed. (c) Effect of a TLR2-blocking antibody on the internalization of α-synuclein into microglia. Primary mouse microglia was pre-incubated with either TLR2-blocking antibody (T2.5) or control (IgG) for 30 min before addition of α-synuclein to the media for 2 h. (d) Ectopic TLR2 expression enhanced uptake of α-synuclein in COS-7 cells. (e) Colocalization of dSY5Y-released α-synuclein with TLR2 in mouse microglia after internalization (top panels).Tlr2−/−mouse microglia show markedly reduced uptake (bottom panels). Scale bar, 10 μm. (f) Fluorescence intensities of internalized α-synuclein in microglia (n=3). All data were analysed using one-way analysis of variance. Error bars represent ±s.e.m. **P<0.01; ***P<0.001. ‘n’ represents the number of independent experiments (see the Methods section). Figure 4: Properties of TLR2 as the receptor for cell-released α-synuclein. ( a ) Competition between TLR2 antibody (T2.5) and dSY5Y-released α-synuclein for binding to the surface of BV2 microglia ( n =3). Scale bar, 10 μm. ( b ) Uptake of α-synuclein by WT and Tlr2 −/− mouse microglia. Cells were treated with αSCM for 30 min, and then analysed. ( c ) Effect of a TLR2-blocking antibody on the internalization of α-synuclein into microglia. Primary mouse microglia was pre-incubated with either TLR2-blocking antibody (T2.5) or control (IgG) for 30 min before addition of α-synuclein to the media for 2 h. ( d ) Ectopic TLR2 expression enhanced uptake of α-synuclein in COS-7 cells. ( e ) Colocalization of dSY5Y-released α-synuclein with TLR2 in mouse microglia after internalization (top panels). Tlr2 −/− mouse microglia show markedly reduced uptake (bottom panels). Scale bar, 10 μm. ( f ) Fluorescence intensities of internalized α-synuclein in microglia ( n =3). All data were analysed using one-way analysis of variance. Error bars represent ±s.e.m. ** P <0.01; *** P <0.001. ‘ n ’ represents the number of independent experiments (see the Methods section). Full size image Role of TLR2 in α-synuclein-induced microglia activation in vivo In order to validate the role of TLR2 in vivo , we induced ectopic expression of human α-synuclein in the SN of WT or Tlr2 −/− mice. Adenoviral vectors for expression of human α-synuclein and green fluorescent protein (GFP) were stereotaxically injected into either side of the putamen, respectively, from which viral vectors were transported in a retrograde manner to the cell bodies of dopaminergic neurons in the SN ( Fig. 5a ). The retrograde transport and expression of viral vectors was confirmed by expression of GFP in tyrosine hydroxylase (TH)-positive neuronal cell bodies in the SN ( Supplementary Fig. S10 ). In a control experiment with the GFP vector, about 15% of nigral dopaminergic neurons expressed GFP. In the SN, all the GFP-positive cells were also TH-positive, verifying that only the dopaminergic neurons expressed human α-synuclein, while microglia did not. Expression of α-synuclein in SN neurons of WT mice resulted in increased microglial activation, while GFP expression caused little change in microglia ( Fig. 5b ). Significant correlation was observed between the level of α-synuclein expression in SN neurons and the degree of microglial activation ( r =0.8519, P =0.0035), while the correlation with GFP expression was insignificant ( r =0.5217, P =0.122; Fig. 5e ). In striking contrast, expression of αSCM in SN neurons of Tlr2 −/− mice led to significantly lowered microglial activation compared with WT mice ( Fig. 5b ), and little correlation was observed between neuronal α-synuclein expression and microglial activation ( r =0.0722, P =0.8777; Fig. 5e ). These results provided verification in vivo that neuronal α-synuclein can activate microglia in a paracrine manner through activation of TLR2. 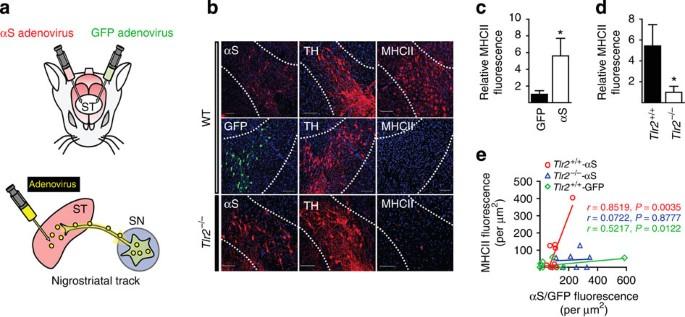Figure 5: TLR2-dependent microglial activation by α-synuclein overexpression in nigral dopaminergic neurons. (a) Experimental scheme. (b) Immunofluorescence images of the SN (dotted lines). Scale bar, 100 μm (c) MHC II fluorescence in the SN of WT mice that received striatal injections of viral vectors expressing GFP and α-synuclein (n=5). (d) MHC II fluorescence in the SN of WT andTlr2−/−mice after striatal injections of α-synuclein vectors (n=5). (e) Correlation between MHC II and GFP/α-synuclein fluorescence in SN (WT;n=9,Tlr2−/−;n=7, GFP;n=12). MHC II fluorescence data (c,d) were analysed using the Mann–WhitneyU-test. Error bars represent ±s.e.m. *P<0.05. ‘n’ represents the number of animals. Figure 5: TLR2-dependent microglial activation by α-synuclein overexpression in nigral dopaminergic neurons. ( a ) Experimental scheme. ( b ) Immunofluorescence images of the SN (dotted lines). Scale bar, 100 μm ( c ) MHC II fluorescence in the SN of WT mice that received striatal injections of viral vectors expressing GFP and α-synuclein ( n =5). ( d ) MHC II fluorescence in the SN of WT and Tlr2 −/− mice after striatal injections of α-synuclein vectors ( n =5). ( e ) Correlation between MHC II and GFP/α-synuclein fluorescence in SN (WT; n =9, Tlr2 −/− ; n =7, GFP; n =12). MHC II fluorescence data ( c , d ) were analysed using the Mann–Whitney U -test. Error bars represent ±s.e.m. * P <0.05. ‘ n ’ represents the number of animals. Full size image Cell-released α-synuclein is a conformation-sensitive agonist of TLR2 We then compared α-synuclein proteins released from dSY5Y cells and proteins residing in the cytosol after purification of these proteins from culture medium and cell lysate, respectively ( Supplementary Fig. S11 ). The cytosolic α-synuclein is mostly monomeric under the denaturing gel condition, whereas the released protein preparation contains significant amounts of stable oligomers ( Supplementary Fig. S11a ). The released α-synuclein, but not the cytosolic protein, activated microglia in a TLR2-dependent manner ( Supplementary Fig. S11b ), and consistently, only the released α-synuclein resulted in TLR2-dependent reporter gene expression, but not the TLR4-reporter gene expression, in a dose-dependent manner in HEK293 reporter cell systems ( Supplementary Fig. S11c,d ). These results suggest that α-synuclein proteins released from cells possess specific modification(s) and/or type(s) of assembly that are essential for becoming the agonist for TLR2. Previous studies have shown microglial activation by various forms of bacterially expressed recombinant α-synuclein proteins [19] , [20] , [21] , [22] . In order to assess the molecular forms of α-synuclein that act as the ligand of TLR2, we tested the following forms of recombinant α-synuclein proteins: monomers, fibrils, oligomers induced by incubation with 4-hydroxy-2-nonenal and mixture of aggregates formed from nitrated α-synuclein ( Supplementary Fig. S12a ). All of the treated forms of recombinant α-synuclein proteins showed much less potency (>30-fold) in cytokine gene induction than αSCM containing a similar quantity of α-synuclein ( Supplementary Fig. S12b ). More important, recombinant α-synuclein proteins showed the same degree of cytokine gene induction in Tlr2 −/− mouse microglia as that observed in WT microglia, suggesting that microglial responses triggered by these forms of recombinant α-synuclein proteins do not involve activation of TLR2. Consistently, recombinant α-synuclein fibrils did not require TLR2 for internalization into microglia ( Supplementary Fig. S13a ), nor did they colocalize with TLR2 after internalization ( Supplementary Fig. S13b ). During the fibrillation, various quasi-stable oligomeric intermediates appear. To assess the role of these oligomers in TLR2 activation, we took samples during the oligomerization of recombinant α-synuclein and evaluated the ability to activate TLR2 in the HEK293 reporter cell system. TLR2 activation was increased over time as the protein aged, but before the appearance of fibrils ( Fig. 6a , Supplementary Fig. S14 ), suggesting that oligomerization was required for α-synuclein to become the agonist for TLR2. To directly address the role of oligomerization, the aged α-synuclein preparation was subjected to the size exclusion chromatography (SEC). ELISA and western blotting clearly showed separation of oligomer, dimer and monomer ( Fig. 6b ). TLR2 activation was observed only in the oligomer fractions (fraction 8 has the highest activity), but not in the dimer or monomer fractions ( Fig. 6b ). Depletion of α-synuclein from the fraction 8 resulted in elimination of TLR2 activation ( Supplementary Fig. S15 ). Oligomers in the fraction 8 were stable in the denaturing gel ( Fig. 6b ), were efficiently recognized by Fila-4 antibody (specific for β-sheet-rich α-synuclein oligomers and fibrils [23] ; Fig. 6c ) and showed a circular dichroism spectrum typical of β-sheet-rich proteins ( Fig. 6d ). Consistent with the reporter assay data, α-synuclein oligomers in fraction 8 interacted with the HEK-Blue-TLR2 cells, whereas the monomers in fraction 14 did not ( Fig. 6e ). Furthermore, oligomers in fraction 8, but not the monomers in fraction 14, efficiently competed with the TLR2 antibody for binding to the microglial cell surface receptor ( Fig. 6f ). 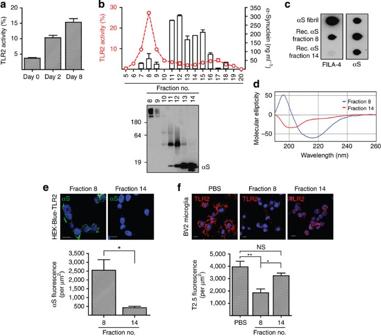Figure 6: Conformation-sensitive agonist activity of α-synuclein for TLR2. (a) Development of TLR2 agonist activity with endotoxin-free recombinant α-synuclein byin vitroincubation (n=3). (b) Separation of ‘aged’ recombinant α-synuclein by SEC. The line trace and the bars indicate TLR2 activity and the α-synuclein levels, respectively. (c) Dot blot analysis of fractions fromb. (d) CD spectra of fractions 8 and 14 fromb. (e) Binding of pure α-synuclein oligomers (fraction 8) on the surface of HEK293 cells expressing human TLR2/CD14 (n=3). (f) Competition between TLR2 antibody (T2.5) and pure preparation of oligomeric α-synuclein for the binding to the surface of BV2 microglia (n=3). Binding data of α-synuclein oligomers (e) were analysed by unpairedt-test. TLR2 fluorescence data (f) were analysed using one-way analysis of variance. Error bars represent ±s.e.m. *P<0.05; **P<0.01. ‘n’ represents the number of independent experiments (see the Methods section). NS, not significant. Figure 6: Conformation-sensitive agonist activity of α-synuclein for TLR2. ( a ) Development of TLR2 agonist activity with endotoxin-free recombinant α-synuclein by in vitro incubation ( n =3). ( b ) Separation of ‘aged’ recombinant α-synuclein by SEC. The line trace and the bars indicate TLR2 activity and the α-synuclein levels, respectively. ( c ) Dot blot analysis of fractions from b . ( d ) CD spectra of fractions 8 and 14 from b . ( e ) Binding of pure α-synuclein oligomers (fraction 8) on the surface of HEK293 cells expressing human TLR2/CD14 ( n =3). ( f ) Competition between TLR2 antibody (T2.5) and pure preparation of oligomeric α-synuclein for the binding to the surface of BV2 microglia ( n =3). Binding data of α-synuclein oligomers ( e ) were analysed by unpaired t -test. TLR2 fluorescence data ( f ) were analysed using one-way analysis of variance. Error bars represent ±s.e.m. * P <0.05; ** P <0.01. ‘ n ’ represents the number of independent experiments (see the Methods section). NS, not significant. Full size image We then asked whether TLR2 activation by dSY5Y-released α-synuclein is mediated by oligomeric forms. Proteins in αSCM were separated with SEC, and each fraction was subjected to α-synuclein ELISA, western blotting, and TLR2 activation assay in the reporter cell system. The highest activity for TLR2 activation was present in the fraction 8, suggesting that dSY5Y-released α-synuclein oligomers are the effective agonist for TLR2 ( Fig. 7a ). In contrast to recombinant monomers and dimers, dSY5Y-released α-synuclein monomers and dimers were capable of TLR2 activation, although their activities were weaker than those of oligomers ( Fig. 7a ). dSY5Y-released α-synuclein oligomers are reactive to Fila-4 antibody, indicating high β-sheet content ( Fig. 7b ). When injected into the cerebral cortices of WT mice, these oligomers (fraction 8 of αSCM) induced microglial activation ( Fig. 7c ). Saline injection into the other hemisphere showed very little microglial activation ( Fig. 7c ). When the same material was injected into the cerebral cortices of Tlr2 −/− mice, neither α-synuclein oligomers nor saline injection resulted in significant activation of microglia ( Fig. 7c ). Monomers/dimers (fraction 14) derived from αSCM are also capable of activating microglia in the cerebral cortices of WT mice, albeit to a much weaker extent ( Fig. 7c ). This activity too disappeared in Tlr2 −/− mice ( Fig. 7c ). This is consistent with the weak activity detected from these monomer/dimer fractions in the TLR2 reporter cells. Therefore, although the majority of TLR2 agonist activity of cell-released α-synuclein is associated with oligomeric forms, a small fraction of monomers/dimers might have either specific modification or conformation that is required for TLR2 activation. Taken together, α-synuclein is a conformation-sensitive endogenous agonist for TLR2; the majority of TLR2 ligand activity resides in β-sheet-rich oligomers among the heterogeneous forms of neuronal cell-released α-synuclein proteins. 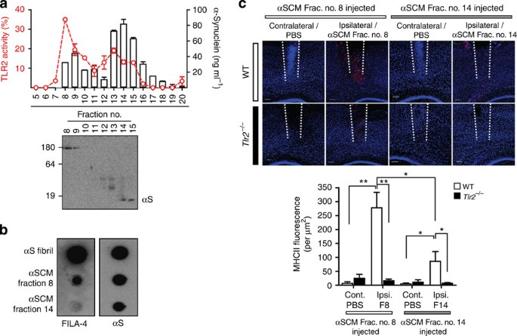Figure 7: Conformation-sensitive agonist activity of cell-released oligomeric α-synuclein for TLR2. (a) Separation of αSCM by SEC. The line trace and the bars indicate TLR2 activity and the α-synuclein levels, respectively. (b) Dot blot analysis of fractions froma. (c) MHC II fluorescence in the cerebral cortices of WT andTlr2−/−mice after injections of fraction 8 and fraction 14 froma(n=5). Data were analyzed using unpairedt-test. Error bars represent ±s.e.m. *P<0.05; **P<0.01. ‘n’ represents the number of animals. Figure 7: Conformation-sensitive agonist activity of cell-released oligomeric α-synuclein for TLR2. ( a ) Separation of αSCM by SEC. The line trace and the bars indicate TLR2 activity and the α-synuclein levels, respectively. ( b ) Dot blot analysis of fractions from a . ( c ) MHC II fluorescence in the cerebral cortices of WT and Tlr2 −/− mice after injections of fraction 8 and fraction 14 from a ( n =5). Data were analyzed using unpaired t -test. Error bars represent ±s.e.m. * P <0.05; ** P <0.01. ‘ n ’ represents the number of animals. Full size image TLR2 upregulation in Lewy body diseases and α-synuclein transgenic mice Paraformaldehyde-fixed vibratome sections from the temporal cortices of human subjects (DLB patients and non-demented control subjects) and sagittal brain sections of mice (α-synuclein transgenic and control mice) were immunolabelled with a TLR2 antibody and analysed for levels of optical density. In control cases, TLR2 antibody mildly labelled pyramidal neurons in the neocortex in layers 2–3 and 5, and some occasional glial cells with morphological characteristics consistent with microglia ( Fig. 8a ). In the DLB cases and α-synuclein transgenic mice, there was a significant increase in the levels of TLR2 immunoreactivity in microglial cells. Upregulation of TLR2 in microglial cells was confirmed by double immunofluorescence studies with antibodies against TLR2 and Iba-1, showing colocalization of the two markers ( Fig. 8b ). This colocalization was seen in most of Iba-1-positive microglial cells, and TLR2 immunofluorescence was stronger in α-synuclein transgenic mice than in control non-transgenic mice. Western analysis also showed significant increases in TLR2 expression in brain homogenates of DLB cases and α-synuclein transgenic mice ( Fig. 8c ). The molecular weight for the mature TLR2 is between 100–110 kDa, and it appears as a doublet. This might represent post-translational modifications such as glycosylation [24] . For quantification, we analysed the doublet, which was bracketed in Fig. 8c . 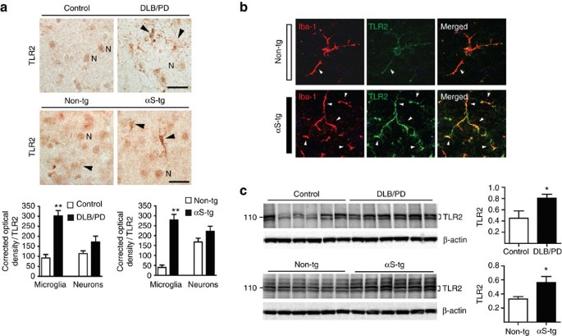Figure 8: TLR2 expression in DLB and α-synuclein transgenic mice. (a) Immunohistochemical analysis of human (top panels,n=6) and mouse samples (bottom panels,n=6). The TLR2 antibody-immunolabelled neuronal cells (N) as well as microglial cells (arrow heads). (b) Double immunofluorescence studies with antibodies against TLR2 and Iba-1 showing colocalization of the two markers in microglial cells (top panels). Double labelling for TLR2 and α-synuclein in the α-synuclein transgenic mice (bottom panels). (c) Western analysis of brain homogenates. All data were analysed using unpairedt-test. Error bars represent ±s.e.m. *P<0.05; **P<0.01. ‘n’ represents the number of patients and animals. Figure 8: TLR2 expression in DLB and α-synuclein transgenic mice. ( a ) Immunohistochemical analysis of human (top panels, n =6) and mouse samples (bottom panels, n =6). The TLR2 antibody-immunolabelled neuronal cells (N) as well as microglial cells (arrow heads). ( b ) Double immunofluorescence studies with antibodies against TLR2 and Iba-1 showing colocalization of the two markers in microglial cells (top panels). Double labelling for TLR2 and α-synuclein in the α-synuclein transgenic mice (bottom panels). ( c ) Western analysis of brain homogenates. All data were analysed using unpaired t -test. Error bars represent ±s.e.m. * P <0.05; ** P <0.01. ‘ n ’ represents the number of patients and animals. Full size image Analysis of transcriptome data from postmortem SN of human PD patients [25] , collected from the public database (NCBI GEO, accession code GSE7621), shows significant increases in expression of genes in the TLR2 signalling pathways, including TLR2, CD14, IRAK2 and NFκB ( Supplementary Fig. S16 ), suggesting that the TLR2 signalling pathway is activated in PD. Our work exemplifies the power of a computational approach for identification of receptors and signalling pathways that are relevant to neurodegenerative diseases. The hypothetical signalling network that we constructed proved to be consistent with experimental results, which demonstrate that cell-released α-synuclein is an endogenous agonist for TLR2 through which microglia are activated and become neurotoxic. The fact that microglial activation by neuronal α-synuclein overexpression in the SN was eliminated in Tlr2 -deficient mice provided in vivo verification of the role of TLR2 in α-synuclein-induced microglial activation. These results implicate a novel mechanism by which neuronal α-synuclein proteins mediate the pathogenic interaction between neuron and glia as a paracrine factor, thereby cultivating inflammatory milieu in brain parenchyma. Our study suggests that elimination of interaction between neuron-released α-synuclein and TLR2 dampens inflammatory responses in the brain, and therefore may be applicable to therapy ( Supplementary Fig. S16 ). Indeed, our recent study suggested that the clearance of extracellular α-synuclein was the mechanism underlying the protective effects of immunotherapy [26] . Recently, a paper by Letiembre et al . [27] reported TLR2 upregulation in several animal models of neurodegenerative disease, including models for AD and PD/DLB, and argued that this response is part of a nonspecific neuroinflammatory effector phase rather than a disease-specific event. We do not intend to argue that TLR2 activation is a specific event in Lewy body diseases. What is disease-specific might be how this pathway is activated. Novelty of our study is that pathogenic protein aggregates that have previously been thought to be confined within neuron can act as an endogenous agonist for the TLR2 pathway. In a recent signalling network analysis, we have hypothesized that cell-released α-synuclein also activates inflammatory responses in astrocytes, including TLR2 activation [8] . This needs experimental validation. We have conducted the uptake and cytokine induction experiments with Tlr2 −/− microglia and the TLR2-blocking antibody, and the cytokine induction was always completely inhibited, whereas the uptake was only partially blocked. Our interpretation is the following: when microglia are exposed to α-synuclein that is secreted from neuronal cells, inflammatory activation of microglia is mediated solely by TLR2, whereas the uptake can be mediated not only by TLR2 but also by other cell surface proteins, such as the scavenger receptors [28] , with the latter being inert in terms of inflammatory signalling. Most of the experiments in our study were conducted at relatively high α-synuclein concentrations (0.1–5.3 μg ml −1 ), compared with the concentrations reported in the cerebrospinal fluid (45–75 ng ml −1 ) [29] and interstitial fluid (up to 8 ng ml −1 ) [18] . However, as shown in Supplementary Fig. 7 , a cytokine induction can be achieved in microglia as low a concentration as 5 ng ml −1 , and TLR2 activation in the reporter system at 1 ng ml −1 (TLR2 reporter system is more sensitive than the assays for microglial responses). At these low concentrations, the responses are very weak but, nevertheless, statistically significant. We do not believe that these weak responses are pathogenic. However, given the fact that α-synuclein secretion is promoted by several factors that are associated with disease, the concentrations used in our study might probably be pathophysiologically relevant. Increased expression of α-synuclein is associated with PD and leads to increased secretion of α-synuclein in neuronal culture [6] . Oxidative stress, defects in protein degradation systems and mitochondrial dysfunction are also strongly associated with PD and promote α-synuclein secretion [5] . Moreover, cytoplasmic calcium can increase the secretion of α-synuclein [30] , raising the possibility that α-synuclein release is regulated by neural activity. Therefore, the concentration of α-synuclein in the interstitial fluid can vary locally and temporarily, and those used in the current study is likely to be within the range of physiological relevance, especially in pathological situation. Several studies have suggested that oligomeric aggregates are the toxic culprit of protein aggregation-associated neurodegenerative diseases [31] . Our study expands the scope of pathogenic functions that oligomeric protein aggregates exert in the pathogenesis of these diseases, by showing that α-synuclein oligomers, through activation of TLR2, are inducers of inflammatory innate immunity in the nervous system. Activation of TLR2 by α-synuclein is highly sensitive to the conformation of the protein; purely monomeric and fibrillar α-synuclein cannot activate TLR2. Oligomerization itself is not sufficient for TLR2 activation; certain types of oligomers, such as the ones induced by HNE, cannot activate TLR2. HNE-induced α-synuclein oligomers generated in our laboratory have little secondary structure [32] , whereas the oligomer preparation that can activate TLR2 showed β-sheet-rich conformation. In addition, the monomer/dimer fractions from αSCM, but not the same fractions from the recombinant α-synuclein, showed a weak TLR2-activating activity, suggesting that there might be certain modification and/or conformation of monomer/dimer occurring in cells that are required for TLR2 agonist activity. Therefore, elucidation of structure of neuron-released α-synuclein is of great importance in terms of understanding of molecular details underlying the interaction between α-synuclein and TLR2. One of the central questions in neurodegenerative diseases is whether inflammatory responses promote neurodegeneration or whether insufficient immune responses contribute to disease. Studies assessing this question have yielded conflicting results. Likewise, whether TLR signalling exacerbates neurodegeneration or is protective in disease progression is still largely unknown. In relation to our current study, more specific question would be whether TLR signalling is hyperactivated by protein aggregates or guide the clearance of protein aggregates. TLRs may mediate the clearance of extracellular protein aggregates. AD mouse models with depletions in TLR genes showed increased cognitive impairments and Aβ deposition [12] , [14] , whereas conflicting results have also been reported; deletion of coreceptor for TLR2/4, CD14 [33] , and a common adaptor protein, MyD88 [34] , ameliorates Aβ deposition. In mice overexpressing mutant SOD1, transplantation of MyD88-deficient bone marrow cells resulted in earlier disease onset and shorter life span that of WT cells [35] . On the other hand, there is a large body of evidence for the role of TLR-mediated neuroinflammation in the initiation and progression of neurodegenerative diseases. Aβ fibrils activated TLR2 and TLR4, and induced inflammatory responses in cultured microglia and monocytes [11] , [15] . TLR4-dependent neuroinflammation was also demonstrated in mouse models of AD [36] . TLR4-activated microglia became neurotoxic [13] and trigger neurodegeneration in mice [37] . In models of SOD1-ALS, TLR-dependent microglial activation exacerbated motor neuron degeneration [38] . TLR3 agonists induced nigral dopaminergic degeneration, which was reversed by systemic administration of an interleukin (IL)-1 receptor antagonist in adult rats [17] , suggesting that TLR activation and subsequent inflammation is disease-promoting. In contrast to the study in the ALS mouse model, transplantation of MyD88-deficient bone marrow cells reduced inflammatory activation and brain Aβ burden, and improved cognitive function in a mouse model of AD [39] . A recent study by Stefanova et al . [40] suggested that TLR4 is involved in α-synuclein clearance in transgenic mice expressing this protein specifically in oligodendrocytes; the same group, however, suggested in an earlier work that microglial activation mediates neurodegeneration in the same mouse model [41] . We speculate that these two seemingly opposite effects of TLRs may not be mutually exclusive. Although the primary role of microglia and its receptors for protein aggregates may be to clear the toxic proteins and protect neurons, microglial responses to TLR activation may change in diseased brains. The outcome of TLR activation may depend on various factors, such as the states of microglial cells, the source and assembly state of protein ligand, duration and strength of the stimulation, and repertoire of coreceptors and adaptor proteins that interact with TLR. The model proposed in the current study ( Supplementary Fig. S17 ) allows the prediction that drugs that act on TLR2 and/or on the extracellular α-synuclein oligomers might modify neuroinflammation in α-synuclein-related neurodegenerative diseases; thus, both these proteins are candidates for mechanism-based drug targets of PD and other related diseases. Of particular interest, other cytosolic aggregation-prone proteins, such as tau and superoxide dismutase 1, are also released from cells [42] , [43] . Moreover, in human tauopathies and the related animal models, neuronal accumulation of hyperphosphorylated tau was closely associated with microglial activation [44] . These results along with those of our current study point to an interesting possibility that microglial activation by neuron-originated aggregation-prone proteins might be a general mechanism of neuroinflammation in major neurodegenerative diseases. Antibodies and chemicals Protease inhibitor cocktail, lipopolysaccharides and DCF-DA were purchased from Sigma-Aldrich (St Louis, MO). Pam3CSK4 and QUANTI-Blue were obtained from InvivoGen (San Diego, CA). The following antibodies were used: TLR2 (clone T2.5) and MHC class II (eBioscience, San Diego, CA); polyclonal TLR2 antibody (US Biological, Swampscott, MA); IκB, p38 MAPK, phospho-p38 MAPK and α-synuclein (polyclonal) (Cell Signaling Technology, Beverly, MA); β-actin (Sigma-Aldrich); nitrated α-synuclein, α-synuclein (LB509), tyrosine hydroxylase and TLR2 (Abcam, Cambridge, MA); α-synuclein (Syn-1; BD Bioscience, San Diego, CA); Iba-1 (Wako Laboratories, Richmond, VA); and FILA-4 antibody (Dr Poul Henning Jensen, University of Aarus). Animals Sprague–Dawley rats and C57BL/6 mice were purchased from Samtako (Osan, Korea). TLR2-deficient mice were obtained from Oriental Bioservice (Kyoto, Japan) [45] , TLR3-deficient mice from R. Flavell (Yale University, School of Medicine, New Haven, CT) [46] and TLR4-deficient mice from S. Akira (Hyogo College of Medicine, Hyogo, Japan) [47] . Transgenic mice expressing WT human α-synuclein under the PGDF-B promoter (line D) were described elsewhere [48] . Genotypes of mice were analysed by PCR using specific primers ( Supplementary Table S3 ). Cell culture Maintenance and differentiation of SH-SY5Y human neuroblastoma, primary cortical neurons, rat and mouse primary microglia, BV2 murine microglial cell lines and COS-7 cells have been previously described [49] , [50] . Polymerase chain reaction Total RNAs were reverse transcribed using the iScript cDNA synthesis kit (Bio-Rad, Hercules, CA). For conventional reverse transcriptase PCR, the complementary DNA products were amplified using specific primers over the indicated cycles ( Supplementary Table S3 ). For real-time PCR, target genes were amplified using SYBR Premix ex taq II (Takara, Shiga, Japan) with specific primers ( Supplementary Table S3 ). Amplification of DNA products was measured by the 7500 Real-Time PCR system (Applied Biosystems, Foster City, CA). Relative mRNA levels were calculated according to the 2 −ΔΔCT method. All ΔC T values were normalized to glyceraldehyde-3-phosphate dehydrogenase or β-actin. Preparation of conditioned media Differentiated SH-SY5Y cells were infected with adenoviral vectors (serotype Ad5, CMV promoter) [51] at a multiplicity of infection of 100. On day 2 post infection, media were replaced with serum-free Dulbecco’s modified Eagle’s medium, then incubated for 18 h. For conditioned media of cortical neurons, mouse cortical neurons were seeded onto 60-mm culture dish. After a 5-day incubation, media were replaced with B27-free neurobasal media, then incubated for 24 h. To remove cell debris, the media were centrifuged at 10,000 g for 10 min. The recovered supernatants were concentrated using 10K cutoff centrifugal filters (Millipore, County Cork, Ireland). Morphological analysis of microglia Microglia cells were treated with CM or lipopolysaccharide for 24 h. Cells with amoeboid and ramified morphologies were counted in ten randomly chosen areas for each experiment, and mean values were obtained. Nitric oxide and cell viability assays Microglia cells were treated with CM or lipopolysaccharide. After a 24-h incubation period, nitric oxide was measured from the microglial culture media using the Griess reagent system (Promega, Madison, WI) according to the manufacturer’s instruction. Cell viability was determined from the cells in the same culture using the Cyquant cell proliferation assay kit (Invitrogen, Carlsbad, CA). Measurement of intracellular reactive oxygen species Microglia cells were treated with 2′,7′-dichlorodihydrofluorescein diacetate (DCF-DA) for 20 min in the dark. A total of 10,000 cells were analysed using a FACSCalibur flow cytometer (Becton Dickinson, Franklin Lakes, NJ). The oxidized form of DCF-DA was excited at 488 nm and detected at 530 nm. α-Synuclein pull down Owing to its affinity to metal ions, α-synuclein binds to the Talon metal affinity resins (Clontech, Mountain View, CA; data not shown). For removal of α-synuclein from αSCM, αSCM was mixed with Talon metal affinity resins and incubated at 4 °C for 2 h with rotation. To isolate cell-released and cytosolic α-synuclein (see Supplementary Fig. S10 ), His-αSCM and cell extracts obtained from dSY5Y cells expressing His-tagged α-synuclein were pulled down with Talon metal affinity resins. Preparation of cell and tissue extracts, and western blot analysis Cells were lysed in the RIPA buffer (150 mM NaCl, 1% Triton X-100, 1% sodium deoxycholate, 0.1% SDS and 50 mM Tris–HCl) with a protease-phosphatase inhibitor mixture. Brain homogenates were prepared in the lysis buffer (1% Triton X-100, 10% glycerol, 50 mM HEPES, pH 7.4, 140 mM NaCl, 1 mM EDTA, 1 mM Na 3 VO 4 , 20 mM β-glycerophosphate and proteinase inhibitor cocktails), and separated into cytosolic and particulate fractions by centrifugation. Western blot analysis was performed as described previously [51] . Tumor-necrosis factor-α and IL-6 measurements The concentrations of tumor-necrosis factor-α and IL-6 were determined by the BIOSOURCE Immunoassay kit (Invitrogen). Microarray experiment and network analysis Microarray analysis was performed on rat primary microglia. RNA preparation, microarray experiment and probe annotation were performed as previously described [8] . Using the normalized intensities, the DEGs (false discovery rate ≤0.01) between LZCM- and αSCM-exposed cells were determined using a previously reported statistical method [8] . For the gene expression data from 9 normal donors and 16 patients with PD (GSE7621), we used the same method to identify the DEGs between normal and patients (false discovery rate ≤0.05). In addition, KEGG pathways enriched by the DEGs were identified ( P <0.01) using DAVID software. For network analysis, we selected a set of DEGs involved in the major pathways and then reconstructed a network describing their interactions and associated pathways based on the interaction data from public databases including BIND, HPRD, BioGRID and KEGG [8] . Analysis of TLR2/α-synuclein interaction The entire procedure was performed on ice in a cold room. BV2 microglia cells were pre-incubated with conditioned medium or SEC fractions for 30 min, then crosslinked by incubation with 2 mM dithiobis(succinimidylpropionate). After the incubation, cells were incubated with either T2.5 (20 μg ml −1 ) or with IgG (20 μg ml −1 ). At least 120 cells were analysed in each independent experiment. For α-synuclein cell surface binding to the HEK293 reporter cells, the cells were incubated with the SEC fractions 8 or 14 for 1 h. At least 220 cells were analysed in each independent experiment. α-Synuclein uptake assay Primary microglia cells were treated with αSCM. After PBS washes, cells were lysed with the Laemmlie sample buffer. In cases of α-synuclein fibril uptake, microglial cells were treated with α-synuclein fibrils (400 nM) and lysed with 1% TritonX-100/PBS. The Triton-insoluble pellets were resuspended in the Laemmlie sample buffer. For ectopic expression of TLR2, COS-7 cells were transfected with pcDNA3.1/Hygro-human TLR2 or with control pcDNA3.1 using lipofectamine 2000 (Invitrogen). Acid washing was performed with 0.1 M HCl twice before lysis. Immunofluorescence microscopy for cells The procedure for immunofluorescence and image analysis have been described elsewhere [52] . Stereotaxic injection and analysis of tissue samples The experimental protocols were approved by Konkuk University’s Animal Care and Use Committee. Adenoviral vectors were prepared using the virakit (Virapur, San Diego, CA). Age-matched mice were stereotaxically positioned under deep anaesthesia, and 1.33 × 10 8 infection units of adenoviral vectors were then injected into striatum (AP; 0.8 mm, ML; 1.7 mm and DV; −3.2 mm). Seven days after injection, the brains were processed for immunofluorescence staining [7] . Immediately adjacent tissue sections were labelled with different antibodies. Fluorescence intensity of unit area measured in the SN region was normalized with that of the non-SN region. Correlation rates were determined by the Pearson product–moment correlation coefficient method (Pearson’s R) using GraphPad Instat software. For the injection of oligomers or monomers, 0.2 ng of αSCM fraction 8 and fraction 14 were injected into the cerebral cortex (AP; 2.0 mm, ML; 1.5 mm, and DV; −1.5 mm). Fluorescence intensity of unit area was measured in the cerebral cortex region around the injection site and normalized with the data obtained from the hippocampus. Preparation of recombinant α-synuclein and aggregates Bacterial endotoxins were removed using the Toxineraser endotoxin removal kit (Genscript, Piscataway, NJ; <0.015 endotoxin unit per 1 mg of α-synucein). Fibrils were prepared as described previously [53] . Nitrated α-synuclein aggregates were generated following the previously described procedure [54] . For HNE-induced oligomerization, α-synuclein (1 mg ml −1 ) was incubated with 1.4 mM HNE (Cayman Chemical, Ann Arbor, MI) for 1 week at 37°C and dialysed against PBS. For spontaneous oligomerization, lyophilized recombinant α-synuclein was dissolved in PBS (1 mg ml −1 ) and incubated at 4°C. After 2 days of incubation, protein was filtrated through a syringe filter with the pore size of 0.2 μm. One hundred microlitres of α-synuclein (50 μM) was separated using Superdex 200 HR 10/30 column (GE Healthcare Life Science) at a flow rate of 0.5 ml min −1 . Circular dichroism Samples (10 μM) were analysed in a Jasco J-810 spectropolarimeter (Tokyo, Japan) from 190–260 nm in a quartz cell at room temperature. The data used for graphical presentation were an average of six different scans. Enzyme-linked immunosorbent assay ELISA was performed as described previously [55] with anti-α-synuclein antibodies Ab62 (1 μg ml −1 ) and biotinylated Ab274 (1 μg ml −1 ) as a capture and reporter, respectively. HEK-Blue TLR reporter assay HEK293 reporter cells stably expressing human TLR2/CD14 and human TLR4/CD14/MD-2 were purchased from InvivoGen along with matching control cells. HEK-Blue TLR reporter assay was performed according to manufacturer’s instructions. Human specimens, neuropathological evaluation and criteria for diagnosis Autopsy material (six non-demented controls and six DLB cases) was obtained from patients studied neurologically and psychometrically at the Alzheimer Disease Research Center/University of California, San Diego ( Supplementary Table S4 ). The last neurobehavioral evaluation was performed within 12 months before death and included Blessed score, Mini Mental State Examination and dementia-rating scale [56] . The diagnosis of DLB was based in the initial clinical presentation with dementia followed by parkinsonism and the presence of α-synuclein- and ubiquitin-positive LBs in cortical and subcortical regions [57] . Procedures for immunocytochemistry and confocal microscopy were described elsewhere [7] . Statistical analysis Statistical significances of data were determined using unpaired t -test, one-way analysis of variance, or Mann–Whitney U -test. How to cite this article: Kim, C. et al . Neuron-released oligomeric α-synuclein is an endogenous agonist of TLR2 for paracrine activation of microglia. Nat. Commun. 4:1562 doi: 10.1038/ncomms2534 (2013).